Giant Raman gain in silicon nanocrystals Nanostructured silicon has generated a lot of interest in the past decades as a key material for silicon-based photonics. The low absorption coefficient makes silicon nanocrystals attractive as an active medium in waveguide structures, and their third-order nonlinear optical properties are crucial for the development of next generation nonlinear photonic devices. Here we report the first observation of stimulated Raman scattering in silicon nanocrystals embedded in a silica matrix under non-resonant excitation at infrared wavelengths (~1.5 μm). Raman gain is directly measured as a function of the silicon content. A giant Raman gain from the silicon nanocrystals is obtained that is up to four orders of magnitude greater than in crystalline silicon. These results demonstrate the first Raman amplifier based on silicon nanocrystals in a silica matrix, thus opening new perspectives for the realization of more efficient Raman lasers with ultra-small sizes, which would increase the synergy between electronic and photonic devices. Nonlinear silicon photonics is a technology for implementing various optical functionalities [1] . Silicon offers a variety of nonlinear effects that can be used to process optical signals at speeds of 100 Gbit s −1 and beyond [2] , [3] and to enable broadband electro-optic modulation [4] , [5] , amplification [6] , [7] and wavelength conversion [8] , [9] . The challenge here is to combine optical and electronic functions on the same chip. The advantages of nonlinear silicon photonics are the potentially low cost and high compatibility with CMOS technology. This approach is very attractive as it allows, for example, exploitation of both the high computation capability of electronics and the large communication bandwidth of photonics. Silicon nanocrystals (Si-nc) find applications in high-density flash memories, in sensing and in photonics [10] , [11] . One of the main issues in the studies of low-dimensional silicon is to control its electronic and dielectric properties to develop new device concepts. The reduction of dimensionality has an effect not only on the linear optical properties (emission efficiency and band gap) but also on the nonlinear optical properties, which are usually enhanced [12] , [13] . Stimulated Raman scattering (SRS) is one of the first discovered nonlinear optical effects where a pump laser beam enters a nonlinear medium and spontaneous generation and amplification lead to a beam at a frequency different from the pump [14] , [15] . In bulk semiconductors, lasing by SRS was first discovered in GaP (ref. 16 ). SRS from glass microspheres was also observed using both pulsed and continuous-wave (CW) probe beams [17] . More recently, Raman lasers have been demonstrated in silicon microwaveguides [18] , [19] , [20] , [21] , [22] , [23] . The investigation of SRS at the nanoscale is a growing field of research. There have been a number of fundamental investigations, both experimental and theoretical [24] , [25] , [26] , [27] , [28] . There are some important perspectives for applications, for example, the realization of micro/nano-light sources with improved performance and reduced size. SRS has been reported from a few nanoscale materials. In Ref. 27 , a large Raman gain was obtained from individual single-walled carbon nanotubes by resonant Raman spectra excited at 632.8 nm. The experimental results were explained by both the exceptional nonlinear properties and the efficient electron–phonon interaction in single-walled carbon nanotubes. In Ref. 28 , SRS from GaP nanowires was also investigated by Raman spectra in backscattering configuration. Using CW laser excitation (514.5 nm), evidence of strong nonlinear SRS was obtained from segments of crystalline nanowires with a diameter of 210 nm and with length of about 1 micron. These observations were discussed in terms of theoretical results developed for dielectric cavities. SRS and lasing in random media have also been demonstrated [29] , [30] , [31] . In view of the importance of nonlinear silicon photonics, SRS in Si-nc is an obvious challenge, and this is the main motivation of the present work. We measure the amplification experienced by a probe beam with a wavelength in the C band of telecommunications in a Raman amplifier based on Si-nc embedded in a silica matrix. We observe that the Raman gain increases with the Si-nc concentration and obtain a gain coefficient up to four orders of magnitude greater than that measured for crystalline silicon. Linear optical characterization of the sample The study was performed on a SiO x ( x <2) film deposited on a silica substrate using the molecular beam deposition method. The sample is about 7 cm long and 1 cm wide. The film has the Si concentration varying along the longer dimension of the sample [32] , [33] , that is, one such sample contains areas with different Si concentrations ( Fig. 1 ). The sample was annealed at 1,200 °C in nitrogen atmosphere, which is known to produce Si-nc in this material [32] , [33] . 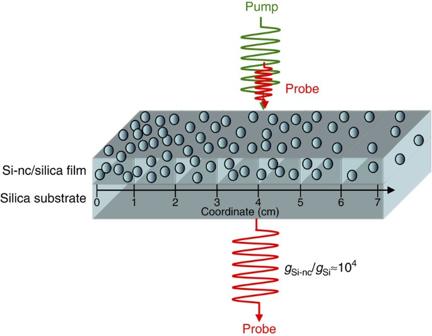Figure 1: Experimental scheme. The film has the Si concentration varying along the longer dimension of the sample, the highest Si concentration being at coordinate 0. The amplification experienced by a probe beam in the presence of a pump beam is measured. Figure 1: Experimental scheme. The film has the Si concentration varying along the longer dimension of the sample, the highest Si concentration being at coordinate 0. The amplification experienced by a probe beam in the presence of a pump beam is measured. Full size image The Raman bands at ~519 cm −1 show the presence of Si-nc in the film ( Fig. 2a ). The Raman bands change in intensity as a function of the coordinate along the longer dimension of the sample, which means that the amount of Si-nc changes accordingly. Transmission electron microscopy suggests sizes of ~4 nm for Si-nc in similar samples [34] . The Si concentration gradient is confirmed by the changes in the absorption coefficient and refractive index ( Fig. 2b ). The film thickness changes as well ( Fig. 2d ). The absorption coefficient and Raman intensity proportionally correlate with each other, increasing with the Si excess. These parameters are known to be proportional to the amount of elemental (‘metallic’) Si measured by X-ray photoelectron spectroscopy (XPS) [35] , [36] . The refractive index also increases with the amount of elemental Si. It should be mentioned that not all the Si excess forms Si-nc seen in the Raman spectra, producing absorption and measured as elemental Si by XPS. A substantial part of Si excess forms Si suboxides and very small Si particles; moreover, a part of the Si particles is amorphous, that is, the Si crystallization is not complete after furnace annealing [35] , [36] . The values obtained for absorption coefficient and refractive index are similar to those measured previously for SiO x films with x from ~1.3 to 1.6 (volumetric proportion of elemental Si from ~10 to 4%) [35] . 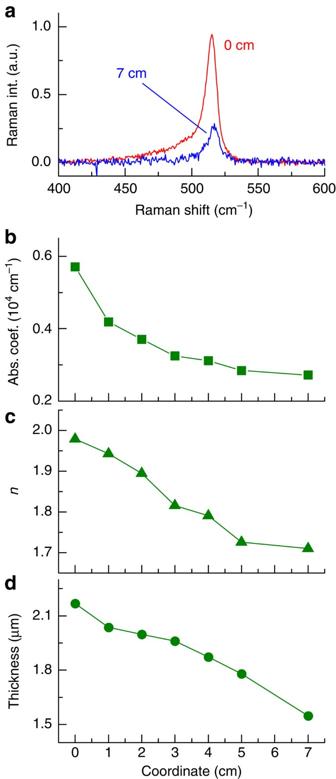Figure 2: Linear optical characterization. (a) Raman spectra of the SiOxsample at the coordinates 0 and 7 cm. The absorption coefficient (Abs. coef.) at 488 nm (b), refractive index (c) and film thickness (d) are shown as a function of the coordinate on the sample. Figure 2: Linear optical characterization. ( a ) Raman spectra of the SiO x sample at the coordinates 0 and 7 cm. The absorption coefficient (Abs. coef.) at 488 nm ( b ), refractive index ( c ) and film thickness ( d ) are shown as a function of the coordinate on the sample. Full size image SRS measurements The film containing Si-nc was mounted perpendicular to the focused pump beam and moved along the Si concentrations gradient ( Fig. 1 ). The experimental set-up is shown in Fig. 3 . We mostly studied six areas with higher Si concentration (coordinates from 0 to 5 cm). 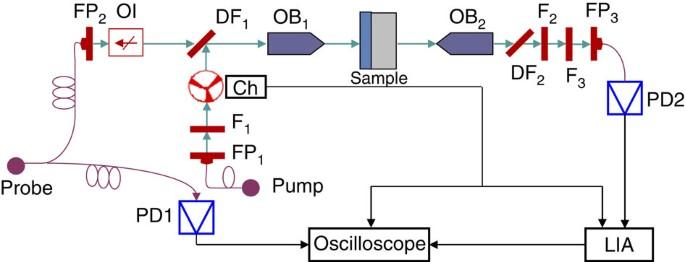Figure 3: Stimulated Raman scattering experimental set-up. Pump, Raman laser; Probe, tunable laser source; FP1and FP2, fibre ports; OI, optical isolator; F1, bandpass filter at 1,427 nm; OB1and OB2, microscope objectives × 50 and × 20; DF1and DF2, dicroic filters; F2, longpass filter at 1,500 nm; F3, longpass filter at 1,460 nm; Ch, chopper; PD1 and PD2, broadband photodetectors; LIA, lock-in amplifier. Black lines represent electrical connections and wiring, green lines represent free-space optical beams and magenta lines represent optical fibres. Figure 3: Stimulated Raman scattering experimental set-up. Pump, Raman laser; Probe, tunable laser source; FP 1 and FP 2 , fibre ports; OI, optical isolator; F 1 , bandpass filter at 1,427 nm; OB 1 and OB 2 , microscope objectives × 50 and × 20; DF 1 and DF 2 , dicroic filters; F 2 , longpass filter at 1,500 nm; F 3 , longpass filter at 1,460 nm; Ch, chopper; PD1 and PD2, broadband photodetectors; LIA, lock-in amplifier. Black lines represent electrical connections and wiring, green lines represent free-space optical beams and magenta lines represent optical fibres. Full size image The Raman gain spectrum is obtained by measuring the fractional change in the probe beam G as a function of the probe laser wavelength (see equation (3) in Methods). As the Raman gain is proportional to the differential cross-section of spontaneous Raman scattering, the Raman gain spectrum should follow the spontaneous Raman spectrum [14] , [15] . In general, accurate measurements of Raman gain spectra are very difficult because relatively small changes in the Stokes signals at different probe wavelengths should be detected. Recently, high-frequency (megahertz) phase-sensitive detection has been successfully employed for single-frequency SRS [37] , although the extension of such measurements to broadband detection is still a challenge [38] . This consideration suggests that our set-up based on amplitude modulation of a CW pump beam is not the best way to measure gain spectra. The shape of the obtained Raman gain spectra is affected by the pump bandwidth and power [39] , [40] , but it is independent of the position on the sample. In fact, we measured Gaussian Raman gain profiles centred at about 519 cm −1 with a width in any case broader than the spontaneous Raman spectra (see Fig. 2a ), which is due to the low spectral resolution of our SRS measurements [41] , [42] . In the SRS measurements, the Raman shift ω p – ω s , where ω p and ω s are the pump and the probe frequencies, respectively, has to match the resonance frequency of a Raman-active mode. To fulfil the matching condition, the spontaneous Raman spectra of Si-nc were used ( Fig. 2a ). For the 1,427 nm pump and the maximum of spontaneous Raman intensity at 519.6 cm −1 , the Raman gain profile is expected to be centred at about 1,541.3 nm. Therefore, in our experiments, the probe wavelength was fixed at 1,541.3 nm. 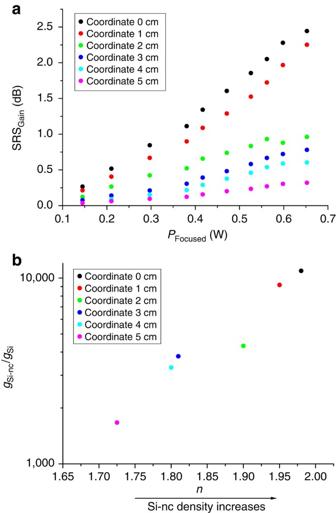Figure 4: Raman gain. (a) Net optical gain of the Stokes radiation (dB) versus the pump powerPFocusedat the sample for different Si concentrations. The area at coordinate 0 cm has the maximum Si concentration. (b) Ratio of the Raman gain coefficients of Si-nc in silica and crystalline silicon as a function of the refractive index of the film with different Si concentrations. Figure 4a presents the net optical gain of the Stokes radiation (SRS Gain ) as a function of the focused pump power measured at the sample ( P Focused ). For the areas with lower Si concentrations (coordinates 6 and 7 cm), the SRS Gain was too small to be accurately measured. For all investigated areas (coordinates from 0 to 5 cm), SRS Gain is a nearly linear function of the pump power (see Fig. 4a ), as expected for the net optical gain of a Raman amplifier. By fitting the SRS Gain data with a linear function and taking into account the film thickness, the Raman gain coefficient g can be obtained (see equation (4)). The Raman gain increases with the Si concentration, which suggests that this phenomenon is connected with the presence of Si-nc. For the sample area with the coordinate 5 cm, we obtain g Si-nc =67 cm MW −1 , whereas for the maximum Si concentration at the coordinate 0, this value is 438 cm MW −1 , which is about four orders of magnitude greater than the value measured for crystalline silicon (see Fig. 4b ). Figure 4: Raman gain. ( a ) Net optical gain of the Stokes radiation (dB) versus the pump power P Focused at the sample for different Si concentrations. The area at coordinate 0 cm has the maximum Si concentration. ( b ) Ratio of the Raman gain coefficients of Si-nc in silica and crystalline silicon as a function of the refractive index of the film with different Si concentrations. Full size image The ‘ideal’ material for Raman amplification should have flat and high Raman gain across a broad wavelength range. However, a tradeoff for Raman amplification is typical: materials with relatively high Raman gain have small bandwidth (for example, silicon), whereas materials with large bandwidth have very small gain (for example, silica). This tradeoff is a serious limitation for the realization of micro- and nano-sources with broad and intense emission spectra. In our previous paper [43] , experimental results on spontaneous Raman scattering in Si-nc at the wavelength of interest for telecommunications (1.54 μm) were reported. We pointed out two significant improvements of silicon quantum dots with respect to crystalline silicon: the broadening of the spontaneous Raman spectra and the tuning of the Stokes shift. Our previous results combined with the present observation of enhanced Raman gain lead us to the conclusion that the traditional tradeoff between gain and bandwidth can be overcome in low-dimensional materials. Most importantly, the present results show an impressive enhancement of the Raman gain in Si-nc compared with bulk silicon, by three–four orders of magnitude depending on the Si concentration (see Fig. 4b ). It should be remembered that the volume of Si-nc does not exceed 10% of the volume of the sample, which makes the difference between the gain properties of Si-nc and bulk silicon even greater. It is also interesting to note that the gain coefficient is not simply proportional to the concentration of Si-nc. The difference of the amount of elemental Si constituting Si-nc increases from coordinate 5 cm to coordinate 0 cm by a factor of about 2, whereas the gain changes by a factor of 6.5. Now, we briefly discuss possible reasons for the giant Raman gain observed from Si-nc. In SRS phenomenon, matter interacts with two light waves at different frequencies (the pump and Stokes waves), where the frequency difference corresponds to the vibrational energy. The origin of SRS can be understood in terms of a two-step process: first, the pump causes the molecular vibrations and thereby produces frequency sidebands (Stokes and anti-Stokes); and next, the Stokes wave beats with the pump wave leading to modulation of the total intensity that coherently excites the molecular vibrations. These two steps reinforce each other in the sense that the pump effect leads to a stronger Stokes wave, which in turn leads to stronger molecular vibrations [14] , [15] . The third-order nonlinear susceptibility is described by χ (3) = χ (3)nr + χ (3)r . The first term, χ (3)nr , represents the non-resonant electronic contribution to the total third-order nonlinear susceptibility, which is a real quantity, and thus is independent of the Raman shift [14] , [15] . This term is related to the nonlinear refractive index (or optical Kerr index) n 2 and two-photon absorption coefficient β . The nonlinear optical properties of Si-nc are affected by their structural parameters (size, distribution, density and crystallinity), and a large variation of the n 2 values has been reported, which complicates the comparison of experimental and theoretical results [44] . Recent studies [45] on nonlinear refractive indices n 2 of SiO 2 films containing Si-nc and/or Si nanoclusters have demonstrated that both the defect states and the quantized electronic states should be taken into account to explain the origin of large values of n 2 of Si clusters, up to two orders of magnitude with respect to crystalline silicon. The second term, the complex quantity χ (3)r , represents the nuclear response of the molecules and provides the intrinsic vibrational mechanism of SRS. It is worth noting that χ (3)r exists only near the vibrational resonance, whereas at the exact Raman resonance χ (3)nr =0 and the Raman susceptibility χ (3)r is negative imaginary, therefore SRS is inherently insensitive to any non-resonant background contributions. Large Raman gain is expected for materials with a large value of Im( χ (3)r ) (refs 14 , 15 ). It has been demonstrated that when the mean-free path of an electron is larger than that of a phonon, the electron can collide with the phonon many times, therefore a strong emission of optical phonons, that is, phonon amplification, can be obtained [27] . From the point of view of energy transfer, the energy of the laser field is first absorbed by the electrons, and then transferred to the phonons through the electron–phonon interaction. We suggest that a similar mechanism may occur in Si-nc. If a resonance condition is obtained, for example, due to the interface levels, and the movement of electrons is strictly restricted due to the confinement effect, all light-generated electrons are expected to be involved in the electron–phonon interaction, resulting in significant amplification of phonons. Therefore, the efficiency of electron–phonon interaction in a nanocrystal may be much higher than in a bulk crystal. Moreover, the structure of interfaces, stoichiometric material disorder, stress and cluster shape may also influence Raman amplification. To better understand our results, a theoretical model of SRS in Si-nc has to be developed, which is outside the scope of our experimental work. In conclusion, a giant Raman gain is obtained from Si-nc in silica, up to four orders of magnitude higher than that from crystalline silicon. From the fundamental point of view, these results will hopefully stimulate theoretical work required to develop a quantitative model of SRS in Si-nc. Concerning applications, we note that the basic idea behind the invention of silicon Raman laser was that the SRS effect in silicon was about 10 4 times larger than that in the glass fibre; therefore, an active device with typical dimensions of a few centimeters instead of several kilometres could be realized. Analogously, according to our results, a Raman laser with a length of a few microns can be developed based on Si-nc. This achievement would lead to all the advantages of combining optical and electronic functions on a single chip. Sample preparation The Si concentration gradient in the sample was achieved by tilting the silica substrate with respect to the silicon beam; hence, the distance from the silicon source to the deposition surface changed across the sample, leading to a variation of the Si flux. Interference patterns were seen by the naked eye from the sample showing gradient of the optical thickness. According to the deposition parameters, the O/Si concentration ratio x was estimated in the present sample from 1.5 (coordinate 0) to 1.8 (coordinate 7 cm). The deposition procedure was previously tested for similar samples using XPS and time-of-flight elastic recoil detection analysis, and these methods systematically showed larger Si concentrations ( x smaller by 10–20%), which is possibly connected with the complex processes of deposition chemistry [35] , [36] . Linear optical characterization The spontaneous Raman spectra were measured with a set-up consisting of an Ar-ion laser (488 nm, Omnichrome 543-AP), a single-stage spectrometer with an optical fibre input (Acton SpectraPro 500I) and a charge-coupled device camera (Andor InstaSpec IV). The film thickness and refractive index were measured using the photoluminescence filtering effect as described elsewhere [33] , [35] . The transmission spectra needed for this procedure were recorded using a fibre-optics spectrometer (SD2000, Ocean Optics) and a broadband light source (DH-2000, Top Sensor Systems). The absorption coefficients at 488 nm were obtained by measuring transmission and reflection of the laser beam. SRS experimental set-up SRS was measured using a Raman fibre laser (IGP Photonics, RLR-5-1427) operating at 1,427 nm as a CW pump laser and a tunable laser source (1,520–1,620 nm, ANDO AQ4321D) as a CW probe laser (see Fig. 3 ). The maximum pump laser power is 5 W and the spectral width (3 dB) is 2 nm. To prepare a collimated pump beam, the output fibre (Corning SMF 28) is connected to a fibre port (FP 1 ). The fibre port (PAF-XM-11-15501) is a miniature micropositioner, providing a stable platform for coupling light into and out of FC/PC- or FC/APC-terminated fibre. A bandpass filter (F 1 , OMEGA 1427BP10) centred at the pump wavelength (1,427 nm) is used to minimize the background. The pump power is measured before the sample by a thermal detector (Gentec PS-310), suitable for high-power CW laser measurement (up to 10 W). In the tunable laser source, an automatic power control circuit is used to maintain very high stability of the output power. However, to take into account possible fluctuations, the probe beam is split by a 1 × 2 fibre-optics splitter (splitting ratio 95/5). The low-power output is used to monitor probe fluctuations by a broadband photodetector (PD1, Thorlabs DET410), whereas the other fibre is connected to a fibre port (FP 2 , PAF-XM-11-15501) to obtain a collimated beam. Amplitude modulation of the pump beam is produced by a chopper operating at 180 Hz. Afterwards, the pump and probe beams are combined by a dichroic mirror (DF 1 , OMEGA 1500DCLP) that transmits longer wavelengths than 1,500 nm and reflects the shorter wavelengths. Subsequently, the two beams are coupled to an infrared long-working distance objective (OB 1 , Mitutoyo M PLAN APO NIR × 50, with numerical aperture (NA)=0.42, working distance=17 mm and focal length=4 mm) to be focused on the sample. The transmitted radiation is collected by an infrared long-working distance microscope objective (OB 2 , Mitutoyo M PLAN APO NIR × 20, with NA=0.40, working distance=20 mm and focal length=10 mm). To separate the probe from the pump, three filters, a dichroic filter (DF 2 , OMEGA 1500DCLP) and two longpass filters, at 1,500 nm (F 2 , OMEGA 1500ALP) and at 1,460 nm (F 3 , OMEGA 1460ALP), are used. The probe signal is measured by a broadband photodetector (PD2, Thorlabs DET410). The signal from PD2 is demodulated by a lock-in amplifier (Signal Recovery, Model 7280 Digital Signal Processing), which is referenced to the chopper. The final acquisition is obtained by a digital oscilloscope (LeCroy Wave Runner 6050) with four channels input. The PD1 output, the chopper analog output and the PD2 analog output channel of the lock-in amplifier are connected to the oscilloscope inputs. The chopper output is used as a trigger, whereas two signals from PD1 and from the PD2 analog output channel of the lock-in amplifier are acquired on a time scale much longer than the lock-in response time. These signals are divided point-by-point and averaged over a large number of acquisitions (10,000), and the averaged value is stored. This measurement is repeated four times and the mean value is analysed, providing the increase of the probe signal as a result of the pump. The accuracy of our measurements of SRS Gain is ±0.1 dB. Loss measurements To suppress Raman gain and to measure the losses at the wavelength used for SRS measurements, the pump was removed and a single beam set-up was used. Losses were obtained by measuring the incident power and the power after the sample. A value of about 0.4 dB was obtained, without a significant dependence on the position on the sample. Raman gain measurements To study Raman gain, the steady-state linear (no pump depletion) regime of SRS can be considered [14] , [15] . In this regime, the intensity of the output Stokes radiation is expressed by where I S (0) is the intensity of the input Stokes radiation, I S ( L ) is the intensity of the output Stokes radiation, I P is the intensity of the pump radiation, g is the Raman gain coefficient and L is the interaction length. When the pump intensity is small, the exponent in equation (1) can be linearized as: In this case, the fractional change in the probe beam G is given by the relation: The Raman gain spectrum is given by the dependence of the fractional change in the probe beam G on the probe laser wavelength. To measure the gain profile, the probe laser wavelength with a bandwidth of 200 kHz was scanned from 1,536 to 1,546 nm, whereas the pump power was fixed at 0.2 W. For high-purity float-zone silicon, we obtained a Gaussian Raman gain centred at about 521 cm −1 with a width in any case larger than 4 cm −1 (Raman spectral width of crystalline silicon) depending on the intensity and bandwidth of the pump beam. Assuming no losses at the Stokes frequency, equation (1) is transformed into where SRS Gain is the net optical gain of the Stokes radiation, I P = P / A , where P is the pump power and A is the effective area of the pump beam. In the case of a thin film, the film thickness represents the effective interaction length. The waist of the pump laser beam was measured by the knife-edge technique, and a value of 5 μm was obtained. The measurements of SRS in silica and high-purity float-zone silicon were carried out. The silica and silicon wafers, with thicknesses 1 mm and 2 mm, respectively, were oriented perpendicular to the focused pump beam. For crystalline silicon, the gain profile is expected to be centred at 1,541.6 nm for the 1,427 nm pump and the 521 cm −1 optical phonon frequency; therefore, to measure the Raman gain in silicon, the probe wavelength was fixed at 1,541.6 nm. When the net optical gain of the Stokes radiation (SRS Gain ) is plotted versus the pump power (measured at the sample), a nearly linear dependence (similar to Fig. 4a ), as expected for the net optical gain of a Raman amplifier, is obtained. By fitting the SRS Gain data with a linear function and taking into account the effective interaction length, the Raman gain coefficient g can be extracted (see equation (4)). For silicon, SRS Gain was reliably observed and the gain coefficient g Si of about 40 cm GW −1 was obtained, in agreement with the experimental values reported previously [46] , [47] , [48] . For silica, we did not find measurable SRS Gain at any probe wavelength; thus, no contribution to the main results from the silica substrate is expected. How to cite this article: Sirleto, L. et al. Giant Raman gain in silicon nanocrystals. Nat. Commun. 3:1220 doi: 10.1038/ncomms2188 (2012).